Atlantic salmon show capability for cardiac acclimation to warm temperatures Increases in environmental temperature predicted to result from global warming have direct effects on performance of ectotherms. Moreover, cardiac function has been observed to limit the tolerance to high temperatures. Here we show that two wild populations of Atlantic salmon originating from northern and southern extremes of its European distribution have strikingly similar cardiac responses to acute warming when acclimated to common temperatures, despite different local environments. Although cardiac collapse starts at 21–23 °C with a maximum heart rate of ~\n150 beats per min (bpm) for 12 °C-acclimated fish, acclimation to 20 °C considerably raises this temperature (27.5 °C) and maximum heart rate (~\n200 bpm). Only minor population differences exist and these are consistent with the warmer habitat of the southern population. We demonstrate that the considerable cardiac plasticity discovered for Atlantic salmon is largely independent of natural habitat, and we propose that observed cardiac plasticity may aid salmon to cope with global warming. Anthropogenic climate change is affecting species distributions and abundance, and adverse ecological effects are predicted to intensify from tropical coral reefs to polar extremes [1] , [2] , [3] . These increases in environmental temperature also have direct effects on performance of ectotherms such as fishes. At the optimum temperature ( T opt ) of fishes the scope for aerobic activity is maximal, and as temperature rises towards sub-optimal temperatures (pejus temperature, T pej ), the aerobic capacity declines because the difference between resting and maximum metabolic rate (aerobic scope (AS)) decreases [4] , [5] . Reduced AS has been linked to reduced growth and reproductive capacity as well as increased vulnerability to predators and diseases [5] , changes that can happen well before AS becomes zero at the critical lethal temperature ( T crit ). Faced with a sub-optimal temperature, a population has the options of either migrating to more suitable environments (if any are available and accessible), acclimating to the new temperature by exploiting its phenotypic plasticity, or adapting through natural selection [6] . Without such responses to climate change, local extinction is inevitable at extreme temperatures [1] . In a variety of fish and invertebrate species, cardiac function has been implicated as a limiting factor for upper temperature tolerance [7] , [8] , [9] , [10] , as indicated by their Arrhenius Breakpoint Temperature ( T AB ) [9] , [10] , [11] , [12] . This is because as the rate of oxygen consumption increases exponentially with temperature, so does the heart rate ( f H ). Moreover, maximum heart rate ( f Hmax ) in fishes ceases to increase at temperatures just beyond T opt , which then puts a limit on the amount of oxygen that can be supplied to tissues above the routine needs [4] , [7] , [8] . Thus, for fishes in vivo (when swimming maximally) and in vitro (pharmacologically stimulated), the rate transition temperatures T AB and T QB (when Q 10 decreases abruptly) for f Hmax have been specifically associated with T opt [11] , [12] . In addition, cardiac arrhythmias develop just below T crit [11] , [12] . Therefore, given its established utility, we used f Hmax to investigate temperature plasticity and tolerance of two wild populations of Atlantic salmon ( Salmo salar ) obtained from the northern (Alta River, Norway, 69°56′N, 23°18′E) and southern (Dordogne River, France, 44°51′N, 0°28′E) limits of its European distribution. By comparing populations naturally separated by a distance of over 3,000 km and inhabiting river systems with very different temperature ranges (~\n3 to 26 °C for Dordogne (ONEMA, Réseau National Thermique, data from 29 October 2000 to 05 June 2009) and −1 to 17 °C for Alta (Norwegian Water Resources and Energy Directorate, Hydrological Department, Hydra II data system, data from 14 September 1980 to 10 September 2007)), we tested the hypothesis that these two populations are locally adapted to their thermal environment. More specifically, we hypothesized that the Dordogne population would have higher thermal tolerance than the Alta population, and warm acclimation would increase the thermal tolerance of the Dordogne population more than the Alta population. To test these hypotheses, eyed eggs from both wild populations were hatched in a salmon nursery (~\n8 °C) at University of Oslo (59°57′N, 10°42′E) and reared from first feeding for ~\n3 months at either 12 or 20 °C before testing the response of f Hmax to warming. This response was used to derive several key rate transition temperatures for f Hmax : (1) T AB , (2) the temperature ( T max ) associated with the highest f Hmax (Max f Hmax ), (3) T QB , which is based on incremental Q 10 values for f Hmax and (4) the temperature when cardiac arrhythmias begin ( T arr ). These functional rate transition temperatures were then compared between populations at two acclimation temperatures. For the most part, the results reject our hypothesis for local adaptation and we show that Atlantic salmon are not tailored to their local biogeography. Independent of the origin, populations have a surprisingly high cardiac capacity to compensate to a warmer than optimal temperature. We suggest that such an attribute may aid Atlantic salmon populations to respond to future warming associated with climate change. Population differences Despite their natural environments being substantially different, both salmon populations shared remarkably similar cardiac responses to acute warming and demonstrated considerable plasticity with temperature acclimation. 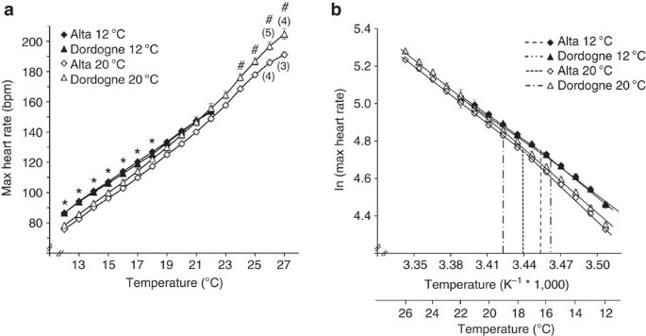Figure 1: The cardiac responses to warming. (a) Average maximum heart rates±s.e. of two populations of Atlantic salmon (Alta,N=5 and Dordogne,N=8 for both acclimation temperatures; otherwise indicated in parenthesis) acclimated to 12 and 20 °C during temperature increase. *Significant difference between acclimation groups;#significant difference between populations (three-way analysis of variance with Holm–Sidakpost-hoctest,P<0.05). (b) Arrhenius plot of maximum heart rate. The dotted vertical lines indicate an Arrhenius break point temperature (TAB) for Dordogne and Alta populations. For example, cardiac collapse at T arr started for both populations at 21–23 °C with 12 °C acclimation, but cardiac remodelling associated with 20 °C acclimation significantly increased T arr to 27.5 °C ( Table 1 ). Therefore, T arr lies well below the critical thermal maxima (CT max ; 32.8 °C with 15 and 20 °C acclimation [13] ). Moreover, for salmon acclimated to 12 °C, significant population differences were absent for any rate transition temperature and associated f Hmax value. Moreover, T max and T arr were always within 0.5 °C of each other, and only 0.8 °C or less separated T AB and T QB ( Table 1 ). Although T arr , T max and Max f Hmax were again similar between populations when they were acclimated to 20 °C, subtle population differences did emerge. For example, T AB for the southern Dordogne population significantly increased with warm acclimation (from 15.7±0.4 to 19.0±0.5 °C), a response not seen in the Alta population (16.4±0.6 versus 17.6±0.6 °C) ( Fig. 1b ). Furthermore, beyond 24 °C the Dordogne population had a significantly higher f Hmax than the Alta population (204.8±3.4 versus 191.2±1.7 beats per min (bpm), respectively, at 27 °C) ( Fig. 1a ), as reflected in the significant 2.5 °C difference in T QB (20.2±0.6 °C versus 17.7±0.7 °C, respectively) ( Fig. 2 and Table 1 ). These subtle differences with 20 °C acclimation are consistent with the southern population being more tolerant of acute warming. Table 1 Heart rate and temperature tolerance differences between populations acclimated to two different temperatures. Full size table Figure 1: The cardiac responses to warming. ( a ) Average maximum heart rates±s.e. of two populations of Atlantic salmon (Alta, N =5 and Dordogne, N =8 for both acclimation temperatures; otherwise indicated in parenthesis) acclimated to 12 and 20 °C during temperature increase. *Significant difference between acclimation groups; # significant difference between populations (three-way analysis of variance with Holm–Sidak post-hoc test, P <0.05). ( b ) Arrhenius plot of maximum heart rate. The dotted vertical lines indicate an Arrhenius break point temperature ( T AB ) for Dordogne and Alta populations. 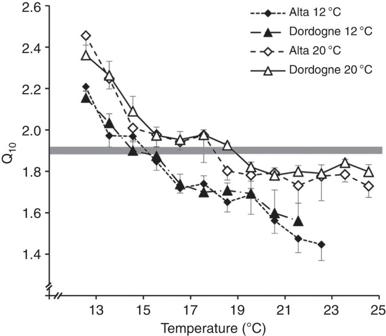Figure 2:Q10changes during warming. AverageQ10±s.e. of maximum heart rate during acute warming of Atlantic salmon (Alta population,N=5 and Dordogne population,N=8 for both acclimation temperatures) acclimated to either 12 or 20 °C. The grey bar (Q10=1.9) indicates the rate transition temperature where maximum heart rate starts an abrupt reduction in its exponential dependence with temperature, which is theQ10break point temperature. Full size image Figure 2: Q 10 changes during warming. Average Q 10 ±s.e. of maximum heart rate during acute warming of Atlantic salmon (Alta population, N =5 and Dordogne population, N =8 for both acclimation temperatures) acclimated to either 12 or 20 °C. The grey bar ( Q 10 =1.9) indicates the rate transition temperature where maximum heart rate starts an abrupt reduction in its exponential dependence with temperature, which is the Q 10 break point temperature. Full size image Effects of temperature acclimation In contrast to the subtle population differences, 20 °C acclimation had a strong effect on f Hmax in both populations. Indeed, at all common temperatures between 12 and 18 °C, f Hmax averaged 8.5±0.7 bpm lower when compared with 12 °C acclimation ( Fig. 1a ). Acclimation to 20 °C also increased Max f Hmax in both populations, reaching ~\n200 bpm at 27 °C compared with ~\n150 bpm at 21 °C with 12 °C acclimation ( Table 1 ). In fact, a difference in acclimation temperature of just 8 °C increased T arr by ~\n6 °C. The cholinergic suppression of f H also appeared to differ between acclimation temperatures ( Table 1 ), as the increase in f H with atropine pretreatment was larger for the 20 °C acclimation groups. Consequently, despite the potential for local cardiac adaptations of juvenile Atlantic salmon due to a spatial segregation of ~\n3,000 km, our results revealed a marked contrast between the considerable cardiac plasticity associated with thermal acclimation and subtle population differences in the thermal performance of the heart. For over a century, wild Atlantic salmon populations have been under significant threat from anthropogenic changes (overfishing, habitat loss, dams, poor water quality), with numerous examples of extinctions [14] . A new, additional threat is climate change, which has the potential to overwhelm the ability of this species to acclimate and/or adapt at the extremes of its biogeographic distribution. Although relocation has been a management solution for other fish species [1] , [6] , salmon have a strong drive to return to their home river for spawning. Indeed, a strong geographic and reproductive isolation is evident in the striking genetic difference discovered between our populations ( Fig. 3 ). Genetic differentiation between Norwegian populations was reported earlier [15] and the Alta population aligns close to those populations. Current thinking is that the diversification among salmonid species and genetic isolation due to anadromy might be connected to climatic cooling during recent ice ages [16] . Moreover, the prevalence of local adaptations increases with geographical distance [17] , which led us to expect local adaption for the Alta population, where the river temperature has not increased above 18 °C for at least the last 30 years, and the Dordogne population, which regularly encounter temperatures over 20 °C in their natural habitat. In contrast to expectations, Alta and Dordogne populations differed very little in their acute cardiac response to temperature, but instead showed considerable cardiac plasticity in response to thermal acclimation that surprisingly was largely independent of the latitudinal and climatic origin of the populations. Therefore, for the most part we rejected the hypotheses of local thermal adaptation in these Atlantic salmon populations. All the same, the Dordogne population had a somewhat higher T QB than the Alta population when acclimated to 20 °C, which seems to suggest a minor but beneficial adaptation to a warmer habitat, despite the two populations responding identically in other aspects to the temperature acclimation. 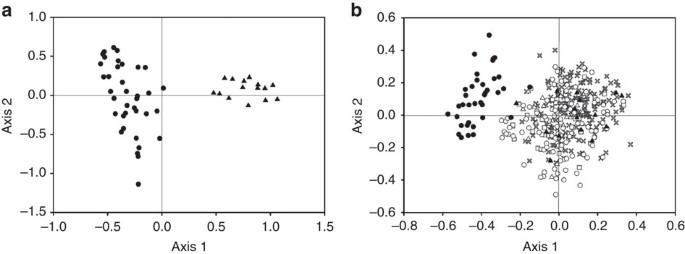Figure 3: Principal coordinates analysis (PCoA) plot based on the genetic diversity among the 14 markers used in this study (GenAlEx 6.5) for population identification. (a) Genetic distance between the Alta (▴) and Dordogne ([cirf ]) populations. Axis 1 and axis 2 explain, respectively, 37.6% and 17.2% of the distribution. (b) Comparison of the genetic diversity observed in the Alta and Dordogne populations, along with other Norwegian populations from Lærdalselva ( × ), Årøyelva (Δ), Suldalslågen (□) and Batnfjordelva (○) (see Johnsenet al.15for location). Axis 1 and axis 2 explain 31.1% and 17.2% of the distribution, respectively. One symbol is one individual,N=52. Figure 3: Principal coordinates analysis (PCoA) plot based on the genetic diversity among the 14 markers used in this study (GenAlEx 6.5) for population identification. ( a ) Genetic distance between the Alta ( ▴ ) and Dordogne ([cirf ]) populations. Axis 1 and axis 2 explain, respectively, 37.6% and 17.2% of the distribution. ( b ) Comparison of the genetic diversity observed in the Alta and Dordogne populations, along with other Norwegian populations from Lærdalselva ( × ), Årøyelva (Δ), Suldalslågen (□) and Batnfjordelva ( ○ ) (see Johnsen et al. [15] for location). Axis 1 and axis 2 explain 31.1% and 17.2% of the distribution, respectively. One symbol is one individual, N =52. Full size image Therefore, the present results emphasize that acclimation remains a feasible possibility for survival in a warmer future, with physiological plasticity replacing the immediate need for local adaptation. If such plasticity enables Atlantic salmon to adequately respond to ongoing warming trends associated with climate change, the southern Dordogne salmon will be physiologically challenged by warming to a greater degree than the northern Alta salmon, because the capacity for cardiac acclimation to warm temperature still resides in the Alta population. The limited local thermal adaptation in Alta and Dordogne salmon populations contrasts with the apparently strong local adaptations revealed for Fraser River adult sockeye salmon ( Oncorhynchus nerka ) populations [8] . The most parsimonious explanation for such a species difference is the athletic requirement of the adult sockeye salmon for its once-in-a-lifetime spawning migration, which has probably been a powerful selective force to optimize AS to local river migration conditions. Such selection may have been relaxed for Atlantic salmon. Consistent with the present study, but on a smaller geographic scale, Norwegian Atlantic salmon populations are known to share similar optimum and critical growth temperatures despite differences in habitat temperatures [18] . Similarly, Arctic char ( Salvelinus alpinus ) populations from Inari, Finland (70°N), and Windermere, UK (54°N), have similar upper incipient lethal temperatures of ~\n23 °C [19] . On the other hand, the thermal acclimation capacity differs among brook trout ( Salvelinus fontinalis ) populations and correlates with habitat temperatures [20] , a similar finding observed among closely related tropical killifishes ( Aphyosemion spp.) [21] and among Danio species [22] , and even among subspecies of the temperate killifish ( Fundulus spp.) [23] . However, some degree of thermal adaptation was discovered after 20 °C acclimation. The southern Dordogne population attained a higher f Hmax above 24 °C and the higher f Hmax was associated with a higher T QB after warm acclimation. Thus, because both T max and T arr were similar between populations, cardiac collapse near T crit would be more precipitous in the southern than in the northern population given the larger difference between T arr and T AB for the northern population. Unexplored here, but still needed, is a consideration of transgenerational changes in temperature tolerance (exposure of parental fish to adverse temperatures providing benefits to offspring) and heritability of thermal tolerance, which can occur in fishes [2] , [24] . Thus, natural selection has the potential to improve thermal tolerance in Atlantic salmon beyond the demonstrated benefits of high thermal plasticity. Also in need of more attention are the cellular responses to both acclimation and warming in different populations because such mechanisms are the proximal cause for differences in organ and whole animal performance. Cellular responses to warming can differ between acclimation temperatures and populations, as shown in redband trout ( Oncorhynchus mykiss gairdneri ) [25] , and may determine whether homeostasis can be maintained at elevated temperatures. Thus, the population differences observed here in Q 10 responses to warming (that is, change in reaction rates) might be associated with important genetic, molecular and enzymatic differences that would need further investigation. The features of cardiac plasticity shared here by both populations are well known in the temperature acclimation literature. In fact, our results are inconsistent with the notion that salmons are stenothermal and have little potential for thermal acclimation [13] . For example, a consistently higher f Hmax at cold temperatures with cold acclimation has been demonstrated for goldfish ( Carassius auratus ) and rainbow trout ( Oncorhynchus mykiss ) (10–20 bpm differences [26] , [27] ). Yet, the 50-bpm shift in Max f Hmax for Atlantic salmon was surprising for an 8 °C acclimation difference, as was the ~\n6 °C shift in T arr . The mechanistic basis for this cardiac plasticity is not fully understood, but is known to include the cardiac sensitivity to adrenaline [28] , the reorganization of sarcolemmal cardiac ion channels [29] and cardiac energy metabolism [12] . The f Hmax obtained here for atropinized and anaesthetized Atlantic salmon at 15 °C (102±1 bpm) was similar to f Hmax measurements in other juvenile salmonids at the same temperature (94 bpm for exercising rainbow trout [30] , ~\n110 bpm for exhausted coho salmon ( Oncorhynchus kisutch ) [11] and ~\n110 bpm for atropine-treated coho salmon [11] ). Therefore, we believe that measuring f Hmax using a pharmacological treatment (atropine) rather than maximal exercise is a reliable surrogate method that avoids several issues related to maximal exercise, including variability induced by stress and behavioural motivation. Indeed, the thermal responses of f Hmax during acute warming have recently been compared between atropinized and exercised fish, and shown to be similar [11] . Moreover, the rate transition temperatures of f Hmax for atropinized fish have been shown to closely relate to thermal tolerance limits in various fish species [11] , [12] , [22] . Thus, upper thermal tolerance limits can be reliably obtained with this method. A limitation to this approach is that a vagal tone may arise due to high temperature triggering a central nervous system response to protect the heart from overload. Such responses have yet to be fully documented, but if they do exist, we would have overestimated the functional upper thermal limits of Atlantic salmon, as do traditional tests of upper thermal tolerance such as CT max tests that use loss of the righting reflex. Another limit of the current study is that without a measurement of resting heart rate, scope for heart rate cannot be calculated. This is likely to be a minor concern given previous studies that show scope for heart rate approaches zero at T opt [4] , [8] and can even become negative at supraoptimal temperatures [8] . Still, further research would be valuable. Although cardiac function is emerging as a particularly important in determining the upper thermal tolerance of a variety aquatic animals [7] , [8] , [9] , [10] , [11] , [12] , many other physiological factors are involved with the overall thermal plasticity of an ectothermic organism. In conclusion, the current study demonstrates that plasticity of maximum cardiac performance of two Atlantic salmon populations is largely dependent on individual thermal history and largely independent of local adaptation when it comes to coping with acute warming. This plasticity might aid northern Atlantic salmon populations to compensate for a warmer future. Experimental animals Eyed eggs originating from wild populations, obtained from Statkraft (Alta population), Norway, and from the Association Migado (Dordogne population), France, were hatched at the University of Oslo (~\n8 °C). From first feeding, the salmon populations were mixed to ensure a similar acclimation treatment and reduce tank effects, and reared for ~\n3 months in two 200-l tanks, one maintained at 12 °C and the other at 20 °C (the animal experiments were approved by the Norwegian Board for Animal Experimentation (approval number 2010/134351)). Fish were fasted for 24 h before f Hmax measurements, which were made during acute warming, a technique first verified for anaesthetized coho salmon to reliably estimate upper temperature limits and T opt (as measured with accompanying AS measurements) [11] . The technique has been subsequently used and verified with other fish species, including rainbow trout [12] and Danio spp. [22] and goldfish [31] . Maximum heart rate measurements Fish ( N =26, sample size was chosen so that statistically significant differences between populations could be evaluated, 3R principle was applied) were weighed and measured before being placed in a sling where they were maintained at anaesthetized state (60 p.p.m. buffered MS-222) while f Hma x measurements were made. Water circulating through the sling, part of which irrigated the gills, was temperature controlled (Hetofrig CB7, Heto, Birkerød, Denmark). Custom-made chromel-A electrodes located underneath the fish and directly below the heart detected a field electrocardiogram, which was amplified (*1,000) and filtered (60 Hz line filter, low-pass 10–30 Hz; high-pass 0.1–0.3 kHz; Grass P55 AC amplifier; Astro-Med Inc., www.astro-med.ca ) and recorded with BIOPAC MP100 data acquisition unit (BIOPAC Systems Canada, Inc., www.biopac.ca ). After a 1-h equilibration period at 12 °C, which allowed heart rate to stabilize, atropine sulphate (1.8 mg kg −1 ) was injected intraperitonally to fully block vagal inhibition of f H . Preliminary tests showed that an isoproterenol injection was not needed to elicit f Hmax at any temperature and the effect of atropine persisted for >10 h. Acute warming (in increments of 1 °C per 6 min) began 15 min after atropine injection. With each 1 °C increment, f Hmax stabilized. Warming continued until the temperature triggered cardiac arrhythmia ( T arr ) when the fish was removed and killed with cranial percussion. A white muscle sample for microsatellite analysis and population identification (see microsatellite analysis paragraph) was then taken and stored at −80 °C. f Hmax was calculated for each 1 °C increment (Acknowledge software version 3.8.1, BIOPAC), which also allowed a calculation of an incremental Q 10 for every temperature step. The Arrhenius breakpoint temperature ( T AB ), which indicates the temperature where a rate functions first fails to follow an exponential increase with temperature [8] , was calculated by plotting natural logarithm of f Hmax against inverse of temperature (Kelvin) and finding best fits for two linear regression lines and calculating their intercept (Sigmaplot 11.0, Systat Software Inc., www.sigmaplot.com ). As f Hmax does not increase with the logarithm function assumed for Arrhenius calculations, especially at high temperatures, T QB indicates the rate transition temperature where the incremental Q 10 for f Hmax abruptly decreases and remains below 1.9 (see Fig. 2 ) and provides another estimate for T opt [12] . Here, T QB was calculated by fitting two segment linear regression lines using the incremental Q 10 as the dependent variable and the temperature increment as the independent variable. Microsatellite analysis After the f Hmax measurements, the individuals were assigned to a population with microsatellite analysis of the white muscle samples [15] . DNA was extracted from frozen white muscle tissue samples (15 samples from fish from Alta and 37 samples from fish from Dordogne) using the E.Z.N.A. DNA tissue kit (VWR, www.vwr.com ) following the manufacturer’s instructions. The average yield reached 11.7 μg of DNA per sample (that is, 58.7 ng μl −1 ). A set of 14 published microsatellite markers ( Table 2 ) was analyzed. Two subsets of seven markers were multiplexed in PCR, using a Multiplex PCR kit (Qiagen, www.qiagen.com ) and the products were run on an ABI 3730 Genetic Analyzer (Applied Biosystems, www.appliedbiosystems.com ). Allele calling was performed in the software GeneMapper v4.0 (Applied Biosystems). FSTAT 2.9.3.2 (ref. 32 ) was used to calculate observed and expected heterozygosity for each marker ( Table 2 ). We used STRUCTURE 2.3.1 (ref. 33 ) to assign individuals to each of two genetic clusters, with the following settings: burn-in length 150,000 followed by 300,000 Markov chain Monte Carlo runs, and no admixture model, that is, individuals were assumed to be discretely from one population or the other. Individuals were assigned to the two clusters with a likelihood of 1 ( Fig. 4 shows the likelihood of group number ( K ) being 2). To visualize the genetic structure, we performed a principal coordinate analysis (GenAlex 6.5). Individuals assigned to each of the two genetic clusters were completely separated in the plot ( Fig. 3a ). To assign genetic cluster to population, we added microsatellite data from four other Norwegian populations to the principal coordinate analysis [15] . One of the clusters of fish from the present study overlapped with the other Norwegian populations ( Fig. 3b ), strongly suggesting that these individuals belong to the Alta population while the other cluster constitutes the Dordogne population. Table 2 Details of the microsatellite loci. 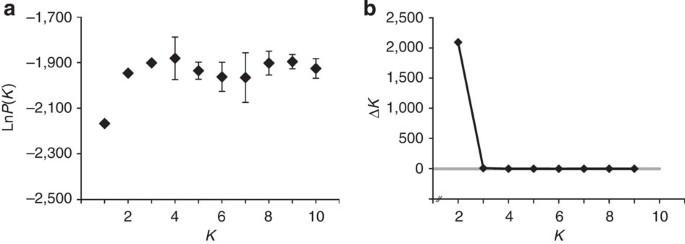Figure 4: Detection of group number (K) in the structure analysis. (a) Mean log-likelihood (LnP(K)±s.d.) for eachK=1–10 and (b) ΔKas calculated with the formula ΔK=mean(|L“K|)/sd[L(K)] (ref.34).N=52. Full size table Figure 4: Detection of group number ( K ) in the structure analysis. ( a ) Mean log-likelihood (Ln P ( K )±s.d.) for each K =1–10 and ( b ) Δ K as calculated with the formula Δ K =mean(| L“K |)/sd[ L ( K )] (ref. 34 ). N =52. Full size image Statistical analyses Based on the population assignment after microsatellite analyses, two-way analysis of variance with Holm–Sidak post-hoc test was used to analyse the differences in body mass, fork length, T AB , T QB , T arr , Max f Hmax , T max and f H before and after atropine injection between populations and acclimation groups. Three-way analysis of variance was used to calculate the differences in f Hmax values at each test temperature between populations and acclimation groups. P <0.05 was considered significant. Values are expressed as mean±s.e. How to cite this article: Anttila, K. et al. Atlantic salmon show capability for cardiac acclimation to warm temperatures. Nat. Commun. 5:4252 doi: 10.1038/ncomms5252 (2014).